Massive gene amplification drives paediatric hepatocellular carcinoma caused by bile salt export pump deficiency Hepatocellular carcinoma (HCC) is almost invariably associated with an underlying inflammatory state, whose direct contribution to the acquisition of critical genomic changes is unclear. Here we map acquired genomic alterations in human and mouse HCCs induced by defects in hepatocyte biliary transporters, which expose hepatocytes to bile salts and cause chronic inflammation that develops into cancer. In both human and mouse cancer genomes, we find few somatic point mutations with no impairment of cancer genes, but massive gene amplification and rearrangements. This genomic landscape differs from that of virus- and alcohol-associated liver cancer. Copy-number gains preferentially occur at late stages of cancer development and frequently target the MAPK signalling pathway, and in particular direct regulators of JNK. The pharmacological inhibition of JNK retards cancer progression in the mouse. Our study demonstrates that intrahepatic cholestasis leading to hepatocyte exposure to bile acids and inflammation promotes cancer through genomic modifications that can be distinguished from those determined by other aetiological factors. Human hepatocellular carcinoma (HCC) arises in response to identifiable causes that in most patients show little or no overlap, including hepatitis C virus (HCV) or hepatitis B virus (HBV) infection, alcohol, exposure to aflatoxin and non-alcoholic steato-hepatitis associated with metabolic diseases [1] , [2] . Because of these distinct aetiologies, the characterization of different types of HCCs allows a basic question in cancer biology to be addressed, namely the specificity of the tumour genomic landscape relative to the disease causative factors. Recent data already suggested that the high genetic heterogeneity of liver cancer depends on the initiating agents. For example, genomic re-sequencing of human liver cancers highlighted recurrent mutations in key cancer genes, such as TP53 and CTNNB1 , and chromatin regulators, but also substantial differences [3] , [4] , [5] , [6] , [7] , [8] . Genes encoding components of the chromatin-remodelling complexes are frequently mutated in hepatitis HCV- but not in HBV-associated HCC [5] . Also the tumour mutational signature (that is, number and type of acquired mutations) strongly depends on the underlying mutagenic mechanism and exposure to different genotoxic chemicals leads to distinct mutation patterns [3] , [4] , [6] . In addition, integration of HBV DNA into the host genome induces genomic instability but may also directly modify cancer driver genes [6] , [8] , [9] , thus triggering oncogenic events. These data clearly show that HCC has a complex pathogenesis in which exogenous factors, inflammation and sustained regeneration cooperate to promote cancer. To understand how liver injury due to a combination of chemical damage, inflammation and fibrosis contributes to the acquired cancer genomic instability, we profiled the genome of human HCCs associated with bile salt export pump (BSEP) deficiency, also known as progressive familial intrahepatic cholestasis type 2. Progressive familial intrahepatic cholestasis designates a heterogeneous group of rare autosomal recessive disorders caused by inherited inactivating mutations in the hepatocyte membrane transporter genes ATP8B1 , ABCB11 and ABCB4 (ref. 10 ). The disease usually appears in infancy or early childhood and manifests with hepatocellular damage and cholestasis due to defects in bile formation [10] . In BSEP deficiency, inherited mutations in the ABCB11 gene cause impairment of bile salt export from hepatocytes into bile, leading to liver chronic inflammation and to the early onset of hepatocellular carcinoma [11] . Thus, this liver cancer type, which we refer to as BSEP-HCC, provides the opportunity to map the acquired genomic modifications that trigger liver cancer in the absence of external mutagenic factors. The genomic profiling of BSEP-HCCs revealed a scenario different from all other HCCs sequenced to date. Exome sequencing showed only very few somatic mutations that did not affect known cancer genes. In contrast, BSEP-HCC genomes acquired massive gene amplification that affected components of signal transduction pathways, such as the ErbB, the PI3K/Akt and the mitogen-activated protein kinase (MAPK) signalling pathways. To further examine the role of these aberrations in cancer onset and progression, we re-sequenced exomes and genomes of HCCs from Mdr2 -KO mice. The Mdr2 -encoded P-glycoprotein belongs to the ABC family of membrane transporters and its absence impairs the secretion of phosphatidylcholine into biliary canaliculi [12] . The resulting high concentration of monomeric bile salts induces hepatocellular damage, inflammation and eventually HCC with high penetrance [13] , [14] , [15] , [16] . It has been suggested that this sequence of events recapitulates to some extent the development of the most common types of human HCCs. In fact, HCCs arisen in chronic liver disease in Mdr2 -KO mice have an aetiopathogenesis similar to that of BSEP-HCCs, while it is clearly distinct from that of viral and metabolic disease-associated human HCCs. Consistent with this notion, in Mdr2- KO HCC we identified very few somatic point mutations, instead we detected a progressive accumulation of gene amplifications affecting the MAPK signalling pathways, and in particular activators of the cJun-N terminal kinases (JNK). Pharmacological inhibition of JNK in the mouse dampened cancer progression. Altogether, our data suggest that the genetic heterogeneity of liver cancers correlates with their distinct pathogenesis and leads to different mechanisms of tumour progression that can be at least partially recapitulated in the mouse. They also provide evidence that solid tumours are not necessarily associated with mutational instability and that, in the specific case of liver cancer, this instability is mostly due to exposure to external mutagens. 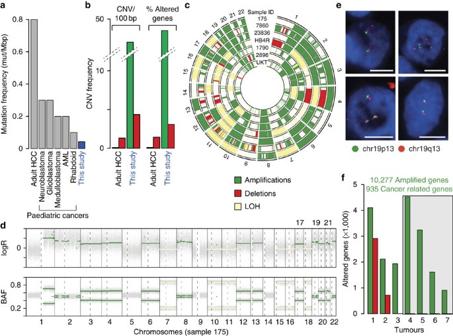Figure 1: Somatic genomic alterations occurring in BSEP-HCCs. (a) Average non-silent mutations frequency in the six BSEP-HCCs as compared with adult HCC and paediatric cancers17. (b) Average CNV frequency in the seven BSEP-HCCs as compared with adult HCC3,6,7. Frequency was measured as CNVs per 100 base pairs and as percentage of altered genes among total human genes. Detailed comparison with each adult HCC screening is reported asSupplementary Fig. 1. (c) Circos plot reporting amplifications, deletions and LOH in all chromosomes of the seven BSEP-HCCs. (d) Copy-number profile of sample 175, as detected from genome wide SNP array. The upper and lower panels show the log ratio of intensity and the B-allele frequency (BAF) of germline heterozygous SNPs, respectively. Amplified, deleted and LOH segments are shown in each chromosome. Dotted lines identify centromeres. (e) Amplification of chromosome 19 in patient 23836 as validated by FISH. Shown are four representative hepatocyte nuclei (blue, DAPI staining) from a paraffin-embedded tumour sample. Probes for chr19p13 (green) and for chr19q13 (orange) were used. Scale bars=20 μm. (f) Amplified (green) and deleted (red) genes in the seven BSEP-HCCs, grouped according to the number of samples in which they were altered. Human BSEP-HCCs do not accumulate mutations in cancer genes To map the somatic mutations acquired in BSEP-HCC, we sequenced the whole exomes of six HCCs and corresponding background livers ( Table 1 and Supplementary Data 1 ). After exome capture, Illumina sequencing and alignment of sequence reads ( Supplementary Data 1 ), we identified a total of 44 single-nucleotide variants (SNVs) and 8 small insertions and deletions (indels) that were present in the six cancer exomes but not in the corresponding background livers (see Methods, and Table 1 ). The orthogonal validation of representative mutations assessed 93% specificity of our variant calling strategy (see Supplementary Methods ). No mutation was shared between any two lesions, and each exome contained on average 0.05 somatic mutations per Mbp ( Table 1 ). This mutation frequency was lower than the average mutation frequency of other human HCCs and of other paediatric cancers [17] ( Fig. 1a ). To exclude the possibility that we did not detect mutations due to poor sensitivity, we measured the false negative rate of the variant calling method at different percentages of tumour content (see Supplementary Methods and Supplementary Table 1 ). We estimated 100% sensitivity in detecting somatic variants in lesions with >40% tumour content. Table 1 Somatic mutations and copy-number alterations in human BSEP-associated liver cancers. Full size table Figure 1: Somatic genomic alterations occurring in BSEP-HCCs. ( a ) Average non-silent mutations frequency in the six BSEP-HCCs as compared with adult HCC and paediatric cancers [17] . ( b ) Average CNV frequency in the seven BSEP-HCCs as compared with adult HCC [3] , [6] , [7] . Frequency was measured as CNVs per 100 base pairs and as percentage of altered genes among total human genes. Detailed comparison with each adult HCC screening is reported as Supplementary Fig. 1 . ( c ) Circos plot reporting amplifications, deletions and LOH in all chromosomes of the seven BSEP-HCCs. ( d ) Copy-number profile of sample 175, as detected from genome wide SNP array. The upper and lower panels show the log ratio of intensity and the B-allele frequency (BAF) of germline heterozygous SNPs, respectively. Amplified, deleted and LOH segments are shown in each chromosome. Dotted lines identify centromeres. ( e ) Amplification of chromosome 19 in patient 23836 as validated by FISH. Shown are four representative hepatocyte nuclei (blue, DAPI staining) from a paraffin-embedded tumour sample. Probes for chr19p13 (green) and for chr19q13 (orange) were used. Scale bars=20 μm. ( f ) Amplified (green) and deleted (red) genes in the seven BSEP-HCCs, grouped according to the number of samples in which they were altered. Full size image Of the 44 somatic SNVs, 15 led to non-silent modifications in 15 genes ( Supplementary Data 2 ). Inspection of these genes pinpointed no strong candidates as drivers of BSEP-HCC. First, none of the mutated genes was a known driver gene in HCC or in any other human cancers [18] , [19] . Second, some of them were known passengers that recurrently mutate in several cancer types [20] , [21] . Finally, most of these genes are either poorly or not expressed in the human liver ( Supplementary Data 2 ), thus indicating that they are probably not functional in this tissue. Overall, our results showed low levels of mutational instability in BSEP-HCC, thus suggesting that the acquisition of mutational instability is not the driving force for the development of this type of liver cancer. Massive gene amplification occurs in human BSEP-HCCs We used genome-wide SNP arrays to investigate the occurrence of copy-number variations (CNVs) in seven BSEP-HCCs, including all tumours screened for point mutations and one additional lesion ( Table 1 ). Compared with adult HCCs, BSEP-HCCs showed higher frequency of CNVs ( Fig. 1b and Supplementary Fig. 1 ), with a total of 18,428, 3,628 and 9,757 genes that underwent amplification, deletion or loss of heterozygosity, respectively, in at least one of the seven samples ( Table 1 and Supplementary Data 3 ). Low-level copy-number gains (on average four copies per aberrant region, Supplementary Fig. 2 , Supplementary Data 3 ) were the most pervasive alterations, with around 38% of the total genome amplified in each sample ( Supplementary Fig. 3A ). We further analysed whether copy-number alterations were focal or arm-level events [22] and observed that deletions were mostly focal and sample specific, except for sample HB4R that had three arm-level deletions involving chromosomes 1p, 4q and 17p ( Supplementary Fig. 3B ). Copy-number gains were instead either arm-level ( Supplementary Fig. 3B ) or multiple focal events that led to the amplification of entire chromosomes, most notably chromosomes 8, 19 and 20 in the majority of lesions ( Fig. 1c,d and Supplementary Fig. 3A ). To validate these results, we performed fluorescence in situ hybridization (FISH) with probes located on both arms of chromosome 19 and confirmed the amplification of this chromosome in sample 23836 ( Fig. 1e ). Multiple amplifications likely occurred via step-wise DNA rearrangements rather than through one-shot catastrophic events, because in most samples we did not detect any sign of chromothripsis. The only exception was sample UKT where several consecutive oscillations between two copy-number states in chromosomes 4 and 6 ( Supplementary Fig. 4A,B , Supplementary Data 3 ) may suggest the occurrence of a one-shot catastrophic rearrangement event [23] , [24] . To find possible cancer drivers, we focused on genes that were recurrently altered in the majority of samples and in particular on 935 known cancer genes that were amplified in the genome of at least four of the seven lesions ( Fig. 1f ). Pathway enrichment analysis of these genes highlighted three top-scoring pathways, namely the MAPK, the ErbB and the PI3K/Akt pathways (corrected P =3 × 10 −06 , 9 × 10 −06 and 2 × 10 −05 , respectively, hypergeometric test, Supplementary Data 4 ). These pathways form a complex and interconnected signalling network [25] , [26] , and their activation is a known driver event in some types of liver cancer [27] , [28] , [29] . The results of the copy-number analysis showed that BSEP-HCCs are characterized by a pervasive occurrence of chromosomal rearrangements that lead to massive gene amplification. Recurrent events involve the amplifications of signalling genes, thus suggesting that the alteration of signalling pathways may be involved in the development and progression of this type of HCC. Mdr2- KO HCCs resemble the genomic landscape of BSEP-HCCs To validate the potential contribution of the genomic modifications in BSEP-HCC, we profiled the cancer genomes of Mdr2 -KO mice, which, similarly to human BSEP-deficient patients, develop HCC due to impairment of bile secretion [12] , [15] . 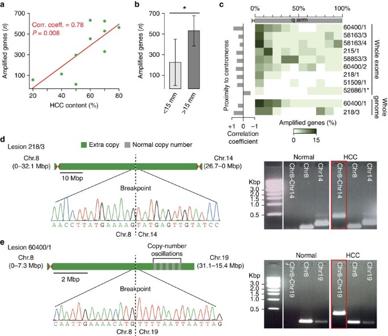Figure 2: Copy-number variations and complex structural rearrangements inMdr2-KO HCCs. (a) Correlation between the number of amplified genes and HCC content in mouse tumours that underwent whole-exome and whole-genome sequencing. Correlation coefficients were measured using the Pearson correlation testing. (b) Comparison between number of altered genes in small (<15mm) and big (>15mm) lesions. *=P<0.05, Wilcoxon test,N=10. Minimum and maximum number of altered genes in the two groups are shown. (c) Cumulative fractions of gene amplifications (amplified genes/total genes) in regions representing 10% of the q arm-length in all mouse chromosomes. In case of exome re-sequencing, the chromosome length was calculated as the region from the first to the last targeted base in the SureSelect XT Mouse All Exon kit (Agilent). Pearson correlation coefficients were calculated between the fraction of amplified genes in each region and the proximity to the centromere of each chromosome. *52686/1 was the only tumour with a negative correlation, likely due to overall CNV underestimation in this sample (see alsoTable 2). (d) Inverted translocations between chromosomes 8 and 14 of lesion 218/3 and (e) chromosomes 8 and 19 of lesion 60400/1. Through the analysis of discordant sequencing read pairs, breakpoints of both rearrangements were mapped at base pair resolutions and confirmed by PCR amplification and Sanger sequencing of breakpoint regions. In sample 60400/1, 10 consecutive copy-number oscillations at chromosome 19 were detected in proximity of the rearrangement with chromosome 8. The genomic coordinates of amplified regions in each chromosome are shown in parentheses. We sequenced the exomes of nine HCCs extracted from the livers of seven Mdr2 -KO mice using the kidney of one of them as a reference ( Table 2 ). We applied the same procedures as those used with human samples for target enrichment, Illumina sequencing and variant calling ( Supplementary Data 5 ) and identified a total of 118 somatic SNVs and no indels ( Table 2 ). Also in this case, we confirmed >93% specificity by orthogonal validation of randomly selected variants (see Supplementary Methods ). None of the 118 SNVs was shared between any two tumours, and 60 of them led to modifications in 60 proteins ( Supplementary Data 6 ). As with BSEP-HCCs, no mutated gene was a known driver of HCC or of other cancers [18] , [19] , and only a few of them were expressed in the liver ( Supplementary Data 6 ). We further sequenced the coding exons of 866 mouse orthologues of human cancer genes ( Supplementary Data 7 ) in four additional Mdr2- KO HCCs, using the normal liver as a reference. In this case, we increased the depth of sequencing coverage to further exclude that mutations might have been missed because of high intratumoral heterogeneity ( Supplementary Data 5 ). Again we found no somatic mutations and no small indels in any cancer genes in any of the four samples ( Table 2 ). Table 2 Somatic mutations and copy-number alterations in Mdr2 -KO mice. Full size table To assess whether the massive copy-number alteration observed in BSEP-HCC also occurred in mouse tumours, we developed a novel method to investigate CNVs directly from targeted re-sequencing data. Our procedure was based on the comparison of normalized gene coverage between tumour and reference that led to the identification of tumour-specific copy-number gains and losses (see Supplementary Methods ). In the 13 mouse HCCs, we identified a total of 2,510 altered genes, almost all of which (2,507) were amplified ( Table 2 and Supplementary Data 8 ). Validation of 10 randomly selected amplified genes using TaqMan copy-number assay estimated 70% sensitivity, 93% specificity and 84% accuracy of the method to call amplifications ( Supplementary Table 2 ). 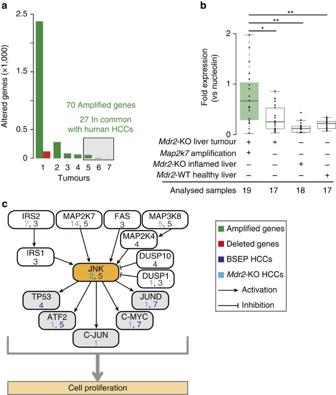Figure 3: Recurrent gene amplifications of JNK interactors in BSEP- andMdr2-KO HCCs. (a) Amplified (green) and deleted (red) genes in all sequencedMdr2-KO HCCs, grouped according to the number of samples in which they were altered. No gene was modified in more than seven tumours. (b)Map2k7expression measured by qPCR inMdr2-KO nodules where the gene was amplified, in nodules with no amplification, inMdr2-KO inflamed livers and in age-matchedMdr2-WT livers. Dots represent the different samples in each group. *=P<0.05, **=P<0.005, Wilcoxon test,N=71. Maximum, minimum and median are shown for each distribution. (c) JNK interactors that are altered inMdr2-KO and BSEP-HCCs. Number of lesions with the amplified gene are reported for mouse (light blue) and human (deep blue). We used genes on chromosome X to assess the performances of our method to detect deletions and estimated 91% sensitivity and 85% accuracy (see Supplementary Methods and Supplementary Table 3 ). We further sequenced the whole genomes of two late-stage Mdr2 -KO HCCs from two different mice, using the corresponding kidneys as matched references. We again observed an overall higher occurrence of amplifications than deletions, with a total of 1,074 amplified and 117 deleted genes in the two genomes ( Supplementary Data 8 ). Since one of the two tumours (ID: 60400/1) had been also used for exome sequencing, we further assessed the performance of CNV detection from targeted re-sequencing data. By far most of the amplified genes detected in the whole exome were also found in the whole genome (85%, Supplementary Data 8 ), thus confirming the reliability of the method. Mdr2 -KO tumours have already been shown to have high degrees of chromosomal instability. In agreement with our results, HCCs from Mdr2 -KO mice that underwent partial hepatectomy show pervasive amplifications, no detectable deletions and recurrent amplifications in chromosomes 5, 8 and 18 (ref. 30 ). Moreover, genes in the 20 Mbps around the centromere of chromosome 8 are upregulated in Mdr2 -KO HCCs [16] . Interestingly, genes in this region were among the most recurrently amplified in our samples (see below and Supplementary Data 8 ). The results of the genomic profiling of Mdr2 -KO HCCs showed that, similarly to human BSEP-HCCs, these tumours are not prone to accumulate somatic point mutations and small indels. Instead, they show pervasive chromosomal instability with overwhelming prevalence of gene amplification. Somatic CNVs accumulate during Mdr2 -KO HCC progression We noticed that human BSEP-HCCs with high tumour content (90%) accumulated more amplifications than those with lower tumour content ( Table 1 ). Interestingly, a positive correlation between tumour size and fold change of the amplified regions was already reported in HCCs from Mdr2 -KO mice that underwent partial hepatectomy [30] . We therefore checked whether a similar signal was detectable in Mdr2 -KO HCCs of our cohort. We indeed confirmed a positive correlation between the number of amplified genes and the HCC content (Pearson’s correlation coefficient=0.78, N =10, Fig. 2a ). Moreover, bigger lesions showed significantly more amplified genes than smaller lesions ( P =0.03, Wilcoxon test, N =10, Fig. 2b ). These results suggested that amplifications tend to occur in larger and more advanced lesions. Furthermore, amplifications preferentially accumulated near the centromeres ( Fig. 2c ) of mouse chromosomes, which are known hotspots for mitotic recombination [31] . Figure 2: Copy-number variations and complex structural rearrangements in Mdr2 -KO HCCs. ( a ) Correlation between the number of amplified genes and HCC content in mouse tumours that underwent whole-exome and whole-genome sequencing. Correlation coefficients were measured using the Pearson correlation testing. ( b ) Comparison between number of altered genes in small (<15mm) and big (>15mm) lesions. *= P <0.05, Wilcoxon test, N =10. Minimum and maximum number of altered genes in the two groups are shown. ( c ) Cumulative fractions of gene amplifications (amplified genes/total genes) in regions representing 10% of the q arm-length in all mouse chromosomes. In case of exome re-sequencing, the chromosome length was calculated as the region from the first to the last targeted base in the SureSelect XT Mouse All Exon kit (Agilent). Pearson correlation coefficients were calculated between the fraction of amplified genes in each region and the proximity to the centromere of each chromosome. *52686/1 was the only tumour with a negative correlation, likely due to overall CNV underestimation in this sample (see also Table 2 ). ( d ) Inverted translocations between chromosomes 8 and 14 of lesion 218/3 and ( e ) chromosomes 8 and 19 of lesion 60400/1. Through the analysis of discordant sequencing read pairs, breakpoints of both rearrangements were mapped at base pair resolutions and confirmed by PCR amplification and Sanger sequencing of breakpoint regions. In sample 60400/1, 10 consecutive copy-number oscillations at chromosome 19 were detected in proximity of the rearrangement with chromosome 8. The genomic coordinates of amplified regions in each chromosome are shown in parentheses. Full size image In the two Mdr2 -KO HCC genomes, we identified inverted translocations involving chromosomes 8 and 14 in one tumour (ID: 218/3, Fig. 2d ) and chromosomes 8 and 19 in the other (ID: 60400/1, Fig. 2e ). Interestingly, mouse chromosome 8 is the ortholog of human chromosomes 8 and 19, which are the most recurrently amplified chromosomes in human BSEP-HCCs ( Supplementary Fig. 3A ). Through the analysis of discordantly aligned read pairs, we were able to map the two breakpoints at base pair resolution and both rearrangements were confirmed with PCR amplification and Sanger sequencing ( Fig. 2d,e ). In one of the two tumours (ID: 60400/1), we counted 10 consecutive disomic and trisomic copy-number states in the region of chromosome 19 involved in the inverted translocation ( Fig. 2e and Supplementary Fig. 3C ). Therefore, again similarly to the human samples, we found possible indications that one-off catastrophic events could be responsible for the acquisition of at least some of the genomic rearrangements in this liver cancer type. In summary, the CNV analysis of Mdr2 -KO HCCs showed that they undergo frequent genomic rearrangements that lead to gene amplifications. Moreover, the observation that CNVs tend to accumulate in large lesions with high HCC content suggests that their putative driver role is exerted in tumour progression rather than in tumour initiation. JNK is deregulated in Mdr2 -KO HCCs Given the similarities in genomic landscapes of acquired alterations between BSEP-HCCs and Mdr2 -KO HCCs, we performed pathway enrichment analysis on 27 genes that were recurrently amplified in both human and mouse cancers ( Fig. 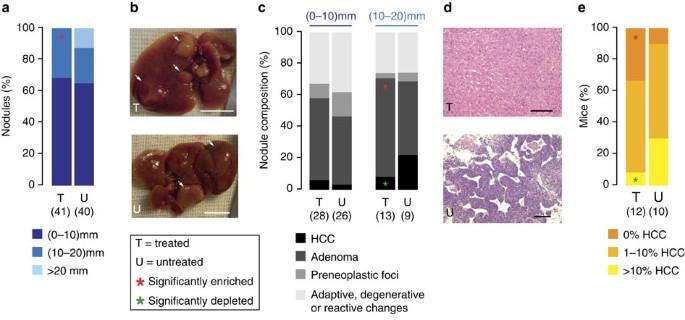Figure 4: Effect of JNK inhibition onMdr2-KO HCC progression. (a) Size differences in nodules from treated and untreatedMdr2-KO mouse groups. Nodules from treated mice were significantly enriched in 10–20 mm lesions, but had no lesions >20 mm. The latter represented ~\n20% of nodules in untreated mice. (b) Representative images of livers from a treated and an untreated mouse. Arrows indicate the nodules. Scale bar=1cm (c) Histological composition of nodules from treated and untreated mice. Nodules in the two cohorts of mice were divided into two groups by size (<10 mm and >10 mm). (d) Representative photomicrographs histologic sections of HCC and adenoma from treated and untreated livers, respectively (hematoxylin/eosin). Scale bar=150 μm. (e) Cumulative tumour content in treated and untreated mice. Tumour content was measured as a percentage of HCC in each nodule. Nodules with HCC fraction >10%, <10% and with no HCC were compared between treated and untreated mice. In all analyses, differences were assessed using Fisher’s exact test. The number of nodules or mice in the two groups are reported in parentheses. 3a , Supplementary Data 8 and Supplementary Table 4 ). Again we found that the MAPK signalling cascade was among the top scoring pathways (corrected P =2 × 10 −02 , hypergeometric test, see Supplementary Methods ). In particular, Map2k7 , encoding the mitogen-activated protein-kinase kinase, was amplified in >70% human and mouse HCCs (5 out of 7 and 10 out of 14, respectively). To better quantify the frequency of Map2k7 amplification, we screened 35 additional tumours from 16 distinct mice using TaqMan copy-number assay. Map2k7 was amplified in 14 of the 49 Mdr2 -KO nodules that were analysed overall (29%, Supplementary Data 9 ), which was a significantly higher proportion than expected by chance ( P =6 × 10 −04 , binomial test). When only nodules with high HCC content were considered, the enrichment became even stronger, with 58% of nodules with ⩾ 40% HCC showing Map2k7 amplification ( P =9 × 10 −05 , binomial test). This result further supports the general observation that gene amplification tends to occur preferentially in lesions with high tumour content ( Fig. 2a ). To investigate whether the additional copies of Map2k7 directly impinge on gene expression, we measured the mRNA levels in tumours where the gene was amplified as compared with tumours where it was not amplified, with Mdr2 -KO inflamed livers and with age-matched healthy livers from Mdr2 -wild type mice. Tumours with Map2k7 amplifications showed significant Map2k7 overexpression compared with all other groups ( Fig. 3b ), thus indicating that gene amplification led to increased expression. Map2k7 specifically regulates the c-Jun NH(2)-terminal kinases (JNKs) [32] , [33] , [34] , which are mainly activated mainly by pro-inflammatory cytokines and environmental stress [35] . Deregulation of JNKs has been already reported to play cell- and stage-dependent roles during HCC development [36] , [37] , [38] , [39] , [40] . Interestingly, upstream and downstream direct JNK interactors, as well as JNKs themselves, were altered in several human and mouse samples ( Fig. 3c ). Figure 3: Recurrent gene amplifications of JNK interactors in BSEP- and Mdr2 -KO HCCs. ( a ) Amplified (green) and deleted (red) genes in all sequenced Mdr2 -KO HCCs, grouped according to the number of samples in which they were altered. No gene was modified in more than seven tumours. ( b ) Map2k7 expression measured by qPCR in Mdr2 -KO nodules where the gene was amplified, in nodules with no amplification, in Mdr2 -KO inflamed livers and in age-matched Mdr2 -WT livers. Dots represent the different samples in each group. *= P <0.05, **= P <0.005, Wilcoxon test, N =71. Maximum, minimum and median are shown for each distribution. ( c ) JNK interactors that are altered in Mdr2 -KO and BSEP-HCCs. Number of lesions with the amplified gene are reported for mouse (light blue) and human (deep blue). Full size image These data showed that gene amplifications occurring in Mdr2 -KO tumours preferentially hit signalling genes, most notably JNK direct interactors or upstream activators, which may have a driver role in triggering liver tumour progression. JNK inhibition arrests carcinoma progression in Mdr2 -KO mice We set out to investigate whether JNK inhibition might interfere with liver cancer progression by treating Mdr2 -KO mice with SP600125, a synthetic polyaromatic chemical that directly inhibits the JNK kinases [41] , [42] , [43] , [44] , [45] , [46] . We randomized 23 Mdr2 -KO mice to receive either SP600125 or vehicle only (12 and 11 mice, respectively, Supplementary Data 10 ). After 3 weeks of treatment, mice were killed and the tumours from the two cohorts were compared in terms of Map2k7 amplification, nodule number, size, histology and tumour content. We found a significantly lower proportion of lesions from treated mice (5 out of 36, 14%) with Map2k7 amplification when compared with lesions from the untreated cohort (13 out of 35, 37%, P =0.03, Fisher’s exact test, Supplementary Data 10 ). Thus, tumours with Map2k7 amplification were more sensitive to JNK inhibition than those without Map2k7 amplification, which explains their relative depletion after treatment. Indirectly, this result also indicated that the effects of SP600125 were mainly caused by its on-target activity on JNK. Moreover, although treated and untreated animals showed a comparable number of tumours per mouse, no mouse treated with the JNK inhibitor had nodules bigger than 20 mm, which instead represented ~\n20% of all lesions in the untreated group ( Fig. 4a,b Supplementary Data 10 ). In a reciprocal manner, the proportion of nodules with diameters between 10 and 20 mm was significantly higher in treated mice than in the untreated group ( Fig. 4a ). Finally, nodules bigger than 10 mm showed significantly higher proportion of adenoma and lower proportion of adenocarcinoma in treated than in untreated mice ( Fig. 4c,d ). No difference was detectable in the histological composition of small lesions (diameter <10 mm). Similarly, treated mice showed an overall significant depletion in HCC, while purely adenomatous nodules were over-represented ( Fig. 4e ). Altogether, these data suggested that the drug blocks tumour progression towards bigger lesions with higher HCC content, thus supporting the role of JNK deregulation in progression more than in initiation of Mdr2 -KO tumours. They were also consistent with the results of the CNV analysis, and specifically with the tendency of gene amplification, and of Map2k7 amplification in particular, to occur in large lesions with high HCC content. Figure 4: Effect of JNK inhibition on Mdr2 -KO HCC progression. ( a ) Size differences in nodules from treated and untreated Mdr2 -KO mouse groups. Nodules from treated mice were significantly enriched in 10–20 mm lesions, but had no lesions >20 mm. The latter represented ~\n20% of nodules in untreated mice. ( b ) Representative images of livers from a treated and an untreated mouse. Arrows indicate the nodules. Scale bar=1cm ( c ) Histological composition of nodules from treated and untreated mice. Nodules in the two cohorts of mice were divided into two groups by size (<10 mm and >10 mm). ( d ) Representative photomicrographs histologic sections of HCC and adenoma from treated and untreated livers, respectively (hematoxylin/eosin). Scale bar=150 μm. ( e ) Cumulative tumour content in treated and untreated mice. Tumour content was measured as a percentage of HCC in each nodule. Nodules with HCC fraction >10%, <10% and with no HCC were compared between treated and untreated mice. In all analyses, differences were assessed using Fisher’s exact test. The number of nodules or mice in the two groups are reported in parentheses. Full size image In this study, we profiled the genomes of aetiologically related mouse and human HCCs to identify the genomic changes acquired in response to chronic exposure to non-neutralized bile acids and in the absence of exogenous direct (viruses) or indirect (alcohol) mutagens. Despite the small sample size that we analysed, our screenings showed a consistent genomic signature within and between species. In both human and mouse, cancer genomes accumulated massive copy-number gain in contrast to very few somatic SNVs or small indels. Such a genomic signature is remarkably different from that of the other HCCs previously sequenced, which acquire mutational instability and tend to accumulate gene deletions rather than amplifications [3] . These findings confirm the genetic heterogeneity of liver cancers caused by different aetiological agents and, at the same time, the remarkable analogy among human and mouse tumours with similar aetiopathogenesis. The detailed analysis of Mdr2 -KO mouse cancer genomes revealed that copy-number gains tend to cluster in genomic regions with high mitotic recombination rates, such as centromeres and telomeres ( Fig. 2c ). These regions are fragile sites prone to rearrangements [47] and are associated with loss of heterozygosity [48] and replication stress [49] , [50] , [51] . Chronic inflammation induces the production of reactive oxygen species that may lead to oxidative DNA damage, thus possibly explaining why genes associated with chromosomal instability are upregulated in the liver of Mdr2 -KO mice [30] , [52] . It is therefore tempting to speculate that recombination hotspots are directly involved in cancer genomic instability in this tumour type, in the absence of external causes of DNA damage. This is also compatible with the role of inflammation in inducing a hypoxic microenvironment that favours chromosomal instability [53] , [54] , [55] . Frequent amplifications of JNK activators, most notably the recurrent amplification of Map2k7 , were found in the majority of mouse and human cancers, suggesting that these modifications may be the driver events in this liver cancer type. Since amplifications of JNK activators preferentially occur at late stages of HCC development, the deregulation of this pathway is likely to favour cancer progression rather than disease initiation. JNK is involved in several physiological and pathological processes including cell proliferation, differentiation, apoptosis and tumorigenesis [35] . Its activation has already been implicated in the development of liver cancer. For example, neither c-Jun nor JNK1 -deficient mice develop HCC after exposure to mutagens [37] , [39] , [40] , [56] . In addition, liver-specific deletion of Mapk14 , a negative regulator of Map2k7 , leads to JNK hyper-activation and HCC development in the mouse [38] . Interestingly, JNK deficiency reduces the onset of inflammation and tumorigenesis when occurring in both hepatocytes and non-parenchymal cells, but it is linked only to increased tumour size when limited to hepatocytes [57] . This hints at an oncogenic role of JNK in non-parenchymal cells where it likely promotes an inflammatory environment that favours transformation and/or tumour progression. Our data support such a scenario, indicating that JNK amplification leads to its deregulation and favours tumour progression in BSEP- and Mdr2 -KO HCCs. In contrast, the JNK pathway is not recurrently amplified in virus-, alcohol- and other risk factor-associated HCCs [3] , [4] , [5] , [6] , [7] , [8] . This further highlights that different disease aetiologies have distinct impacts on tumour genomics, which in turn may lead to different molecular mechanisms of tumour initiation and progression. Since we observed that pharmacological inhibition of JNK impairs the adenoma-to-carcinoma progression in vivo , JNK inhibition may be useful to block HCC onset in BSEP deficiency patients waiting for liver transplantation. In this regard, it is important to notice that the drug used to block JNK (SP600125) has been reported to exert secondary effects on targets other than JNKs [58] , [59] . However, the fact that tumours with Map2k7 amplification were significantly depleted on treatment suggests that the effects of SP600125 were mainly accounted for by the ability to inhibit JNK. In conclusion, this study demonstrates that intrahepatic cholestasis leading to hepatocyte exposure to bile acids and chronic inflammation generates a unique and distinctive signature of genomic changes that can be clearly distinguished from those caused by viruses and other external factors. It will be interesting to determine whether and to what extent similar genomic changes represent a general feature of tumours arising from other chronically inflamed tissues. Human sample description and DNA extraction Samples used in the study were obtained from frozen or formalin-fixed paraffin-embedded (FFPE) material from seven children diagnosed with BSEP-HCC, with parental written consent ( Supplementary Data 1 ). The protocol for use of human tissues was approved by the review board of the corresponding hospital of provenience (French Institute of Medical Research and Health IRB Number 11-047; UK Integrated Research Application System ID: 103273, REC reference:12/WA/0282; Italian Ministry of Health, statement 61, 19/12/1986 N.900.2/ Ag 464/260; Ethical Review Board of the University Hospital Tübingen, Ref.no, 27/2008B01). All specimens were obtained at native-liver hepatectomy during transplantation. The background liver in all patients exhibited parenchymal rather than portal-tract cholestasis, with BSEP expression detectable in none. Some patients had frank cirrhosis, others only fibrosis, which varied in degree from patient to patient ( Supplementary Data 1 ). Samples 7860 175, 1790, 2896 and UKT came from single-unencapsulated masses, while sample 23836 derived from one of several HCC within a single liver. Sample HB4R was a relapse that developed within allograft liver 6 years after transplantation. The patient was treated with chemotherapy before relapse and surgical resection. In all samples, non-neoplastic liver tissues from the same patients were used as matching background references. Genomic DNA was extracted from each tumour from matched background liver tissue using the DNeasy Blood and Tissue Kit (Qiagen) for frozen samples and with the AllPrep DNA/RNA FFPE Mini Kit (Qiagen) for FFPE blocks. Exome sequencing, variant calling and mutation validation Target capture was done on six human tumour and reference samples ( Supplementary Data 1 ) using the SureSelect XT Human All Exon V4 kit (Agilent) targeting 20,965 human genes, following the manufacturer’s protocol with minor modifications. Sample UKT was excluded from whole-exome sequencing because of the low tumour content (see Supplementary Methods ). Around 3 μg of genomic DNA was sheared using an Adaptive Focused Acoustics technology (Covaris). After library preparation with an Illumina DNA Sample Prep Kit, 200 bp fragments were selected using the Agencourt AMPure PCR Purification system (Beckman Coulter). Fragments were further amplified with 5 to 7 cycles of PCR and 500 ng was hybridized with the bait library. DNA capture was followed by paired-read cluster generation on the Cluster Station (Illumina). Libraries were sequenced using one-half lane of Illumina HiSeq2000 per sample, with 76 bp or 101 bp paired-end protocol, except for the tumoral sample of patient 7860, where one entire lane was used due to high levels of DNA degradation ( Supplementary Data 1 ). Paired-end sequencing reads from each tumour and reference were mapped to the human genome (GRCh37/hg19) using Novoalign ( http://novocraft.com ). At most three mismatches per read were allowed and duplicated reads were removed using rmdup of SAMtools [60] . All reads uniquely mapping within 75–100 bp of the targeted regions were considered on target and retained for further analysis ( Supplementary Data 1 ). SNVs and indels were identified using SAMtools [60] and VarScan 2 (ref. 61 ) and retained if covered by at least 10 reads and with frequency ⩾ 20%. Somatic mutations and indels were identified as tumour-specific mutations with coverage ⩾ 5x, frequency <10% in the reference, and not present in dbSNP build 137 (MAF >1%). All 44 SNVs and 8 indels were retained after manual inspection, and 14 non-silent SNVs underwent orthogonal validation (see Supplementary Methods ). Functional annotation of mutated genes The list of genes affected by mutations was intersected with the genes known to be recurrently mutated in HCC ( TP53 , CTNNB1 , ARID1A , ARID2 , AXIN1 , RPS6KA3 , VCAM1 , CDK14 , TERT , MLL4 , CCNE1 ) [18] and with the list of 537 genes known to have a causative role in human cancer [19] . Expression levels of mutated genes in the normal liver were inferred from publicly available data [62] , [63] . Starting from the raw CEL files of the two experiments, data were normalized and analysed using the MAS5 algorithm. The expression level for each gene in the liver was calculated as the mean value among all gene probes with detection P -value <0.05. If all probes of a gene had P -value >0.05, the gene was considered not expressed. The normalized expression level was then measured as the gene expression level over the median expression of all genes in the liver. Genes with expression higher than the median were considered to be high expressed, while all genes with expression lower than the median were defined as low expressed. Recurrently mutated passenger genes were retrieved from literature (refs 20 , 21 and http://bio.ieo.eu/ncg/ ). SNP array and copy-number calling in the human samples Genomic DNA extracted from FFPE samples and from frozen samples was processed according to the Infinium HD assay ultra manual. DNA from FFPE samples was restored before SNP array processing according to the Infinium HD FFPE restore protocol. All seven human tumours and matched background livers were assayed using Illumina HumanOmniExpress-12 v1.0, and image data were scanned using a BeadArray reader. Intensity and genotype data were extracted for CNV analysis after normalizing raw fluorescence signals using Illumina Genome Studio v2011.1. CNV analysis was performed using ASCAT (version 2.1), which takes into consideration aneuploidy and non-aberrant cell admixture present in each tumour sample [64] (see Supplementary Methods ). For six tumours with whole-exome sequencing data, frequency distributions of the germline heterozygous SNPs were integrated with the SNP array results to identify high confidence CNV regions (see Supplementary Methods ). To identify altered genes, the genomic coordinates of the aberrant regions in each sample were intersected with those of 20,965 human genes of the SureSelect XT Human All Exon V4 kit (Agilent). A gene was considered as modified if ⩾ 80% of its length was contained in an aberrant region. Fluorescence in situ hybridization Validation of amplification of chromosome 19 in sample 23836 was performed by two-colour fluorescence in situ hybridization (FISH) using a Vysis LSI 19q13 SpectrumOrange/19p13 SpectrumGreen probe (Abbott), according to the manufacturer’s instructions. Two-micrometre FFPE slides from the tumour and background liver of patient 23286 were deparaffinized in xylene, washed in 100% ethanol, incubated in 1 × SSC (0.3 M sodium chloride, 0.03 M sodium citrate) pH 6.0 at 80 °C for 20 min for demasking and digested with pepsin (0.5 mg ml −1 in 0.2 N HCl, pH 1.0; Protease and Protease Buffer II, Abbott) for 17 min at 37 °C. Samples were then washed in 2 × SSC, dehydrated in 70, 95 and 100% ethanol and air dried. Ten microlitres of probe was directly applied onto each slide and topped with a coverglass that was then sealed with rubber cement. Slides were placed in a HYBrite (Abbott), and the probe was left to denature 1 min at 85 °C, followed by an overnight hybridization at 37°C. Coverglasses were then removed and slides were washed twice in 2 × SSC with 0.1% NP-40 at RT, once in 0.4 × SSC with 0.3% NP-40 at 73 °C and once again in 2 × SSC with 0.1% NP-40 at RT. After counterstaining with DAPI (Sigma), FISH signals were scored with an Olympus BX61 upright microscope, using a × 100 objective. Gene enrichment and pathway analysis Pathway enrichment was done with ConsensusPathDB [65] . A total of 935 human cancer genes amplified in at least four BSEP-HCCs, and 27 genes that were amplified in the majority of human and mouse HCCs, were compared with the pathway-base gene set composed of 10,529 pathway-associated genes. P -values were calculated with the hypergeometric test based on the number of pathway components present in both the amplified cancer gene set and the pathway-base gene set. The resulting P- values were then corrected for multiple testing using false discovery rate. Mouse description and DNA extraction Experiments involving mice have been done in accordance with the Italian Laws (D.L.vo 116/92) and mice have been housed according to the guidelines of the European Commission Recommendation 2007/526/EC—June 18, 2007. The project has been notified to the Italian Ministry of Health (project n. 106/11). Founders of the FVB.129P2-Abcb4 tm1Bor /J ( Mdr2 -KO, stock number: 002539) and FVB/NJ ( Mdr2 wild type, stock number:001800) mice were purchased from The Jackson Laboratory. Colonies of both strains were maintained under specific pathogen-free conditions. Adenoma and HCC nodules from Mdr2 -KO mice were snap frozen for DNA/RNA extraction or fixed in formalin for histological analysis. Initial pathological stage (inflammation) DNA/RNA extraction was carried out on purified populations of hepatocytes obtained via collagenase liver perfusion, using a two-step protocol [66] . The normal livers or kidneys were collected and frozen to be used as reference. Frozen tissue samples were homogenized with a GentleMACS Dissociator (Miltenyi Biotec) before column extraction. Genomic DNA was extracted using the DNeasy Blood and Tissue Kit (Qiagen) according to the manufacturer’s protocol for all samples and matching wild-type tissue. Mouse histology All analysed samples were inspected by a mouse pathologist. Tumour growth in Mdr2 -KO livers is multicentric; grossly detectable masses are often very heterogeneous resulting from the collision of multiple contiguous hepatocellular proliferations with different histologic features and grades. In addition, there is a tendency for hepatocellular carcinoma to develop within an adenoma (as foci of tumour progression). In this context, local invasion (one of the most reliable indicators of tumour malignancy) is difficult to assess and carcinoma diagnosis relies entirely on the recognition of clear features of architectural or cytologic atypia. Given these peculiar characteristics of tumour growth in Mdr2 -KO mice, the histological composition of grossly detectable hepatic nodules was semiquantitatively determined based on reported classification criteria [67] . Selection of the 866 mouse orthologues of human cancer genes A collection of 2,061 human cancer genes was selected from the Cancer Gene Census [19] , COSMIC ( http://cancer.sanger.ac.uk/cancergenome/projects/cosmic/ ) and high-throughput cancer mutational screenings ( http://bio.ieo.eu/ncg/ ). The 1,753 mouse orthologues of these genes were identified using eggNOG [68] and MGI ( http://www.informatics.jax.org ), and only the 866 with RefSeq entries were selected ( Supplementary Data 7 ). The SureSelect Custom kit (Agilent) was designed to capture 15,067 exons of the 866 genes, for a total of 2.7 Mbp of DNA. Exons shorter than 60 bp (except for those with mutations in COSMIC), sequence repeats, segmental duplications, PAR regions and gaps were excluded. Finally, only regions with GC content ranging from 30 to 65% were selected to optimize the capture efficiency. Whole-exome and whole-genome sequencing of mouse samples The SureSelect custom kit was used for the 866 selected genes and the SureSelect XT Mouse All Exon kit (Agilent) was used to target 21,543 mouse genes following the manufacturer’s protocol with slight modifications. In brief, around 3 μg of genomic DNA was sheared using an ultrasonic disruptor (Bioruptor, Diagenode) or using an Adaptive Focused Acoustics technology (Covaris). After library preparation with the Illumina DNA Sample Prep Kit, 200–250 bp fragments were selected and purified by gel extraction, or using the minelute PCR purification kit (Qiagen), or using the Agencourt AMPure PCR Purification system (Beckman Coulter). Fragments were further amplified with 10 cycles of PCR and 500 ng was hybridized with each bait library. DNA capture was followed by single- or paired-read cluster generation on the Cluster Station (Illumina). The libraries obtained for the 866 genes were sequenced on the Genome Analyzer IIx with the 76 single-end protocol, using one lane for each tumour sample or matching normal sample. The libraries obtained for the whole exomes were sequenced using one-half lane of Illumina HiSeq2000 per sample, with the 101 bp paired-end protocol ( Supplementary Data 5 ). For whole-genome sequencing, around 1 μg of mouse genomic DNA was sheared in 400–500 bp fragments using an ultrasonic disruptor (Bioruptor, Diagenode). Libraries were prepared with Illumina Paired-End DNA Sample Prep Kit. The libraries obtained were sequenced using one lane of Illumina HiSeq2000 per sample, with the 101 bp paired-end protocol ( Supplementary Data 5 ). CNVs and structural rearrangements in mouse samples To detect CNVs on targeted re-sequencing data, we developed an in-house pipeline based on the difference in sequencing coverage between tumours and normal counterparts (see Supplementary Methods ). Copy-number analysis on the whole-genome sequencing data was performed using CNVnator v. 0.2.5 (ref. 69 ) (see Supplementary Methods ). Structural rearrangements were inferred using PEMer [70] with slight modifications to adapt the method to Illumina sequencing. Paired-end insert size distribution was calculated to determine the expected insert size range. All mapped paired-end pairs that displayed either an insert size greater than expected or an unexpected orientation were selected. Of these, only discordant read pairs overlapping with or next to mapped CNV regions in the tumour were selected for manual inspection. Identified rearrangements between chromosomes 8 and 14 (ID: 218/3) and 8 and 19 (ID: 60400/1) were confirmed with PCR amplifications and Sanger sequencing. Expression quantitation of Map2k7 Total RNA for qRT-PCR experiments was extracted from Mdr2 -KO tumours, Mdr2 -KO inflamed livers and age-matched Mdr2 -WT healthy livers in Trizol (Invitrogen) using the RNeasy Mini Kit (Qiagen) according to the manufacturer’s instructions. Total RNA (0.5 μg) was used for cDNA synthesis (using ImProm-II Reverse Transcriptase, Promega). Quantification was performed on Nanodrop, and quality was assessed on Bioanalyzer (Agilent). Expression analysis was carried out by qPCR on 1 μl of cDNA reverse-transcribed from 0.5 μg of total RNA. qPCR (SYBR Green, Applied Biosystems) analysis was performed on an Applied Biosystems 7500 Real-time PCR system. Values were normalized for nucleolin content. Treatment with SP600125 JNK inhibitor Twenty-three Mdr2 -KO mice were randomly divided into two groups at the age of 13 to 14 months, when nodules are already formed [15] . One group of 12 mice was treated with an SP600125 (anthra[1,9-cd]pyrazol-6(2H)-one) (Calbiochem), and the other group of 11 mice with vehicle Supplementary Data 10 ). Vehicle for SP600125, diluted in DMSO, was 40% polyethylene glycol (PEG, Sigma) in PBS. Treatments (60 mg per dose) were administered intraperitoneally three times a week for a total of 3 weeks. Mice were killed 1 week after the end of the treatment, and all grossly detectable nodules were counted, measured with a caliper and collected for DNA extraction and histological analysis. How to cite this article: Iannelli, F. et al . Massive gene amplification drives paediatric hepatocellular carcinoma caused by bile salt export pump deficiency. Nat. Commun. 5:3850 doi: 10.1038/ncomms4850 (2014). Accession codes: Exome sequence data for human HCC samples have been deposited in the European Genome-phenome Archive (EGA, http://www.ebi.ac.uk/ega/ ) under the accession code EGAS00001000749. Whole-genome, whole-exome and targeted re-sequence data for mouse HCC samples have been deposited in GenBank/EMBL/DDBJ Sequence Read Archive (SRA) under the accession codes SRP040716 , SRP040691 and SRP040712 , respectively.